Chiral plasmonic DNA nanostructures with switchable circular dichroism Circular dichroism spectra of naturally occurring molecules and also of synthetic chiral arrangements of plasmonic particles often exhibit characteristic bisignate shapes. Such spectra consist of peaks next to dips (or vice versa) and result from the superposition of signals originating from many individual chiral objects oriented randomly in solution. Here we show that by first aligning and then toggling the orientation of DNA-origami-scaffolded nanoparticle helices attached to a substrate, we are able to reversibly switch the optical response between two distinct circular dichroism spectra corresponding to either perpendicular or parallel helix orientation with respect to the light beam. The observed directional circular dichroism of our switchable plasmonic material is in good agreement with predictions based on dipole approximation theory. Such dynamic metamaterials introduce functionality into soft matter-based optical devices and may enable novel data storage schemes or signal modulators. Circular dichroism (CD) of an optically active material describes the differential absorption of left- and right-handed circularly polarized light. The characteristic shape of CD spectra recorded from molecules such as proteins or DNA–usually appearing in the ultraviolet range–reflects their chiral geometry and originates from the superposition of CD signals of many randomly oriented molecules in solution. Surface plasmon resonances in chiral assemblies of metal nanoparticles can also give rise to strong and characteristic CD responses at visible wavelengths [1] , [2] , [3] , [4] , [5] . Manufacturing dynamic plasmonic materials that interact with visible light in a controllable fashion is challenging: a metallic or dielectric substrate must be structured on a length scale smaller than the wavelength of the exciting electromagnetic field. For the visible range this implies a characteristic scale of tens of nanometres, whereas for infrared wavelengths this requirement is relaxed to hundreds of nanometres [6] , [7] . Top-down fabrication methods are readily available for the latter length scale, and therefore remarkable progress has been already achieved for switchable plasmonic materials functioning in the infrared and longer wavelengths [8] , [9] , [10] . Furthermore, to dynamically alter optical responses of metamaterials, generally three approaches can be pursued. First, the electromagnetic properties of the meta-atoms are altered, which can be achieved, for example, by controlling electric currents [11] , [12] , [13] . Second, the electromagnetic properties of the surrounding material are altered. This is equivalent to observing changes in the environment, an approach successfully applied in sensing applications [14] , [15] , [16] , [17] , [18] . Third, changes in the material’s geometry are enabled. This has been shown successfully for micrometre-scale geometries [19] ; however, the control of nanoscale geometries is only possible in a limited way in lithographically produced structures. By using molecular linkers, it is possible to detect shifts of plasmonic resonances in absorption or scattering spectra upon aggregation or spatial reorganization of nanoparticles [20] , [21] . And although absorption and scattering measurements are certainly suitable methods for the detection of frequency shifts, controlled switching of CD spectra of chiral interacting plasmonic objects that are assembled with soft matter templates enables entirely new detection schemes and introduces dynamic behaviour into metamaterial research. For example, recent studies observed the induced emergence of CD signals in solutions during the formation of nanorod aggregates [4] or the self-assembly of nanorod dimers of left- and right-handed chirality [5] . In this Article, with the aim to create a dynamic two-state plasmonic material and to overcome the above-mentioned obstacles, we mount switchable chiral nanostructures that are assembled using the DNA origami method on a glass substrate. The DNA origami method allows the assembly of complex two- and three-dimensional shapes by annealing hundreds of short single-stranded DNA (ssDNA) oligonucleotides with a long ssDNA during a thermo-controlled process [22] , [23] , [24] , [25] , [26] . DNA nanostructures can be precisely decorated with metal particles with nanometre precision [27] , [28] , [29] , [30] , [31] and we and others recently demonstrated the assembly of gold particles into left- and right-handed nanohelices with perfectly controlled chirality [2] , [32] . Notably, these particle helices exhibit strong optical activity, which can be tuned by particle-directed metal deposition [2] , [33] , [34] through a wide range of the optical spectrum. Aligning chiral plasmonic nanostructures on glass surfaces For our experiments, left-handed nanohelices (L-NHs) are attached via bio-linkers to a substrate in a way that they are switchable in orientation ( Fig. 1 ). For the L-NHs, 10 nm gold particles are attached to the surface of a rigid DNA origami 24-helix bundle (24HB) to form a secondary helix with a diameter of 34 nm, a helical pitch of 57 nm and a total length of 79 nm. Each particle attachment site on the 24HB consists of three 15 bases long single-stranded extensions protruding from the DNA origami surface. Previous to assembly, the gold nanoparticles were functionalized with multiple thiol-modified DNA strands ( Fig. 1a ), which are complementary to the staple extensions. These particles were mixed with the assembled 24HBs followed by gel purification to remove unbound nanoparticles. Electron microscopy reveals the formation of the particle helices ( Fig. 1b ). The face at one end of the 24HB was modified with 10 biotin molecules to attach the L-NHs on a BSA–biotin–neutravidin-coated quartz glass surface. Because of the multiple attachment sites and the large area of the DNA structure’s face, the gold helices stand upright as it has also been shown previously with four- and six-helix bundles with broadened ends [35] , [36] . We performed single-molecule measurements to confirm the upright orientation of the gold nanohelices in solution as discussed later. Quartz surfaces coated with nanohelices were placed in a test tube for a step of additional silver growth on the nanoparticles surfaces (metal enhancement). It is worth mentioning that it is also possible to assemble the gold particles on the origami structures after they have been attached to the surface. For this procedure, surface-bound 24HB with bare attachment sites are placed in a solution containing the gold particles functionalized with the sequences complementary to the attachment sites. The gold particle helices assemble within 1 h, no further purification is required and the unbound gold particles can simply be removed with a pipette and later be reused for further assemblies. Another advantage of this method is that only nanohelices that are actually standing upright will offer all their attachment sites for gold nanoparticle binding. 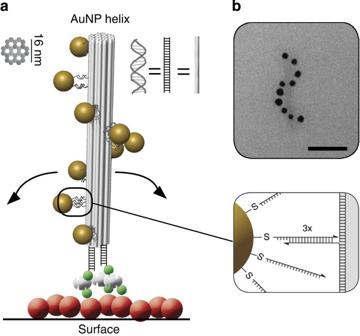Figure 1:Surface-bound chiral plasmonic nanostructure. (a) A rigid DNA origami bundle composed of 24 parallel double helices. Gold nanoparticles are arranged in a secondary left-handed helix on the DNA origami structure. Zoom in: 10 nm gold nanoparticle functionalized with thiolated ssDNA hybridized to the DNA origami 24HB. The origami structure is functionalized with biotin groups (green) on one end for the attachment to a BSA–biotin–neutravidin-coated surface (red, green and grey). (b) Transmission electron microscopy image of a nanohelix adsorbed non-specifically to a carbon-coated grid. Scale bar, 50 nm. Figure 1: Surface-bound chiral plasmonic nanostructure . ( a ) A rigid DNA origami bundle composed of 24 parallel double helices. Gold nanoparticles are arranged in a secondary left-handed helix on the DNA origami structure. Zoom in: 10 nm gold nanoparticle functionalized with thiolated ssDNA hybridized to the DNA origami 24HB. The origami structure is functionalized with biotin groups (green) on one end for the attachment to a BSA–biotin–neutravidin-coated surface (red, green and grey). ( b ) Transmission electron microscopy image of a nanohelix adsorbed non-specifically to a carbon-coated grid. Scale bar, 50 nm. Full size image Switching the CD signal For the CD measurements, the nanohelix-covered quartz glass is placed perpendicular to the measurement light beam inside a buffer-filled cuvette. The nanohelices standing upright on the substrate are hence aligned parallel to the beam ( Fig. 2 ). Owing to the flexibility of the linkers and the roughness of the protein substrate, we did not expect to achieve perfect alignment, that is, all helices standing exactly perpendicular to the surface. Nonetheless, we observed a dominant plasmonic CD signal of left-handed helices when the circularly polarized light passes through the samples along the helical z axis (CD z ). Instead of the peak-dip (bisignate) CD of the L-NHs isotropically dispersed in solution ( Fig. 2a ), an inverted dip-peak spectrum with a dominant peak at the plasmon resonance is expected from theory ( Fig. 2b , see Supplementary Fig. S1 and Supplementary Table S1 for other geometries) and becomes apparent in the experiment at 528±4 nm ( Fig. 2c ). In the next step the quartz glass was dried with nitrogen and placed again into the emptied cuvette. This resulted in the alignment of the L-NHs parallel to the glass surface and therefore perpendicular to the light beam. As expected, the recorded CD spectrum shows a peak-dip signal with a dominant dip at 552±4 nm (CD xy ). The CD xy spectrum is flipped along the horizontal axis and slightly red shifted (24±8 nm) compared with the CD z . The wavelength shift between CD xy and CD z agrees with the calculations for nanohelices in a uniform media. However, it should be noted that the refractive index around the gold nanoparticles could also affect the wavelength shift to some extent (see Supplementary Fig. S2 ). To show the reversibility of the CD switching, the cuvette is filled again with buffer and a new CD spectrum is recorded. Judging from the recovered CD z signal, it can be concluded that the L-NHs stand up again and align parallel to the light beam, although some of the helices or individual nanoparticles may have been washed away and some helices may have stuck permanently to the substrate during the flushing and drying process, respectively (see also Supplementary Fig. S3 ). Another drying step switches the orientation and the CD signal once more. It is hence possible to reversibly switch between two alignment states and subsequently gather the signals of CD z and CD xy without changing the orientation of the substrate (see Supplementary Fig. S4 for switching CD spectra of right-handed nanohelices and Supplementary Fig. S5 for switching CD spectra of L-NHs assembled on the surface). 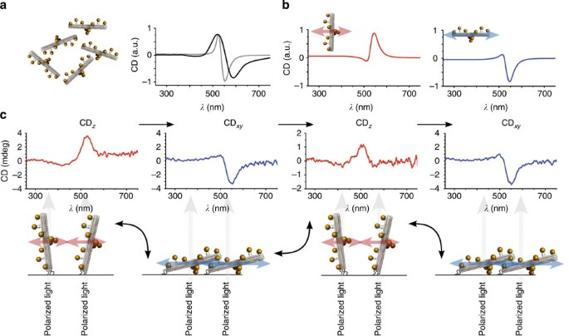Figure 2: Dynamic material with switchable CD. (a) Theoretical (grey curve) and experimental (black curve) CD spectra for L-NHs dispersed in solution. (b) Theoretical CD spectra of L-NHs oriented parallel (red curve) and perpendicular (blue curve) to the incident beam. (c) Experimental CD spectra (top) and scheme of orientation state (bottom) of the L-NHs. The light beam penetrates the quartz substrate perpendicular to its surface plane. Measurements shown were performed with the same ensemble of L-NHs and in the displayed order. L-NHs stood upright if dispersed in solution and were hence aligned parallel to the incoming light beam. The expected transverse CDzwas observed in this case. After removal of the buffer and drying of the surface, the L-NHs laid flat on the substrate and were thus oriented perpendicular to the incoming light beam. Here, the expected longitudinal CDxywas measured. The cuvette was re-filled with buffer, which led to re-alignment of the L-NHs parallel to the light beam. Again the transverse CDzwas obtained. The sample was dried again and the longitudinal CDxyreappeared. Figure 2: Dynamic material with switchable CD. ( a ) Theoretical (grey curve) and experimental (black curve) CD spectra for L-NHs dispersed in solution. ( b ) Theoretical CD spectra of L-NHs oriented parallel (red curve) and perpendicular (blue curve) to the incident beam. ( c ) Experimental CD spectra (top) and scheme of orientation state (bottom) of the L-NHs. The light beam penetrates the quartz substrate perpendicular to its surface plane. Measurements shown were performed with the same ensemble of L-NHs and in the displayed order. L-NHs stood upright if dispersed in solution and were hence aligned parallel to the incoming light beam. The expected transverse CD z was observed in this case. After removal of the buffer and drying of the surface, the L-NHs laid flat on the substrate and were thus oriented perpendicular to the incoming light beam. Here, the expected longitudinal CD xy was measured. The cuvette was re-filled with buffer, which led to re-alignment of the L-NHs parallel to the light beam. Again the transverse CD z was obtained. The sample was dried again and the longitudinal CD xy reappeared. Full size image Our results agree well with theoretical models: the nanohelices dispersed in solution show the aforementioned peak-dip CD spectra in the visible [1] , [2] , [37] , [38] , [39] , [40] , [41] , [42] . This shape can be explained by a splitting between the plasmonic modes in a nanoparticle helix. On the opposite sides of the plasmon peak, the plasmon modes have opposite chiralities and therefore a CD spectrum receives its bisignate appearance ( Fig. 3a ). In addition to the slight frequency shift, the calculation shows that CD of transversely oriented helices results in a peak in the spectrum (for L-NH), whereas the signal of longitudinally oriented helices results in a dip ( Fig. 3b ). As the frequency shift is small, the total CD strength of non-oriented helices is significantly weakened due to the cancellation of CDs from all possible helix orientations. Consequently, an increase of the signal for aligned helices is expected. This increase, however, is strongly dependent upon the variation of orientation–recall the incomplete orientation due to surface roughness and flexibility of the linker molecules–of the nanohelices with respect to the incoming light beam. To account for this effect, we calculated the influence of the angle variation of the standing helices on the CD z ( Fig. 3c ) (see Supplementary Note 1 ). The given angle describes the opening angle of a cone that accommodates all helix orientations. Interestingly, even an opening angle of 70° still allows a dominant CD z to occur. The comparison of these calculations with our experimentally obtained CD spectra in combination with evaluating the density of the aligned L-NHs on a quartz surface by scanning electron microscopy suggests that the cone opening angle might be as large as 60° for our standing helices. Importantly, we find an increase of the CD signal of 3–8-fold for aligned L-NHs over randomly oriented L-NHs in solution (see Supplementary Figs S6–S8 ). Note that substrate-related interferences can influence such measurements and have to be taken into account for quantitative analysis. In our case, however, the effects became negligible in the plasmonic range (above 500 nm, see Supplementary Fig. S9 ). 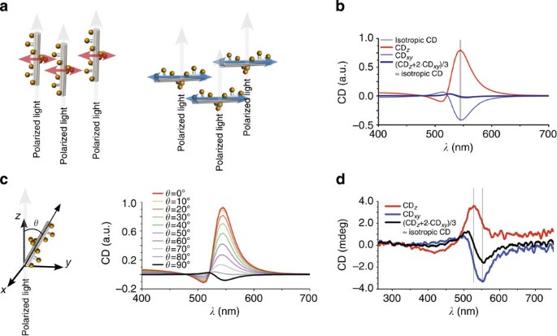Figure 3:CD splitting theory and comparison to experimental results. (a) Scheme of L-NHs aligned orthogonal and parallel to a polarized light beam. The possible CD excitation modes are indicated with double arrows (red, CDz; blue, CDxy). (b) The simulated peak-dip CD signal of randomly oriented L-NHs can be composed by the superposition of weighted transverse CDzand longitudinal CDxysignals. The directional CD signal (CDzor CDxy) is much stronger than the signal originating from randomly dispersed helices as averaging over the orientation of the chiral objects typically strongly reduces the CD signal. (c) Simulated CD spectra for helices oriented at angles restricted to a cone with a given opening angleθ. (d) The CDz(red curve) and the CDxy(blue curve) were measured from the same ensemble of L-NHs by switching the orientation of the L-NHs (cf.Fig. 2). The black curve shows the calculated superposition of weighted CDzand CDxy. Importantly, this curve resembles the CD signal of nanohelices dispersed randomly in solution. Note that the peak shift between the inverted modes (indicated by the grey vertical lines) is larger than expected from theory (as indicated inb). This can be attributed to differences of the refractive indices of the particle-surrounding media in dry and wet samples. Figure 3: CD splitting theory and comparison to experimental results . ( a ) Scheme of L-NHs aligned orthogonal and parallel to a polarized light beam. The possible CD excitation modes are indicated with double arrows (red, CD z ; blue, CD xy ). ( b ) The simulated peak-dip CD signal of randomly oriented L-NHs can be composed by the superposition of weighted transverse CD z and longitudinal CD xy signals. The directional CD signal (CD z or CD xy ) is much stronger than the signal originating from randomly dispersed helices as averaging over the orientation of the chiral objects typically strongly reduces the CD signal. ( c ) Simulated CD spectra for helices oriented at angles restricted to a cone with a given opening angle θ . ( d ) The CD z (red curve) and the CD xy (blue curve) were measured from the same ensemble of L-NHs by switching the orientation of the L-NHs (cf. Fig. 2 ). The black curve shows the calculated superposition of weighted CD z and CD xy . Importantly, this curve resembles the CD signal of nanohelices dispersed randomly in solution. Note that the peak shift between the inverted modes (indicated by the grey vertical lines) is larger than expected from theory (as indicated in b ). This can be attributed to differences of the refractive indices of the particle-surrounding media in dry and wet samples. Full size image To finally illustrate the formation of the commonly observed bisignate CD shapes, the CD spectrum of L-NHs dispersed randomly in solution is recomposed by superimposing two subsequently recorded CD z and CD xy spectra and by giving a weight of one-third to helices oriented parallel to the light beam (CD z ) and two thirds to perpendicularly aligned helices (CD xy ) ( Fig. 3d ). This result is in very good agreement with our theoretical model. Single molecule darkfield scattering spectroscopy In addition to ensemble measurements on oriented helices, also single molecule measurements were performed. To assay the specificity of the nanohelix attachment to the functionalized quartz surface, darkfield microscopy videos of nanohelices before and after the biotin modification were recorded ( Supplementary Movies 1 and 2 ) and to further determine the orientation of nanohelices on the surface darkfield scattering spectroscopy was employed. Our calculations for the scattering show excitation of the transverse plasmon modes for the nanohelices aligned parallel to the light beam and excitation of both the transverse and longitudinal plasmon modes for the nanohelices aligned orthogonal to the light beam ( Fig. 4a ). For our experiments we expected the frequency shift between these plasmon resonances to be 20.5 nm ( Fig. 4b ). 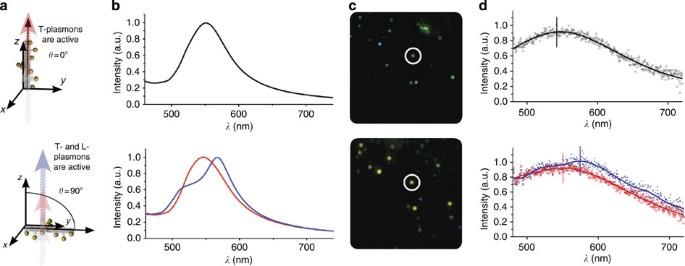Figure 4:Darkfield scattering spectroscopy of surface-bound nanohelices. Aligned nanohelices orthogonal to a surface in solution (top row) and aligned nanohelices parallel to a surface dry on glass (bottom row) were studied. (a) Schemes of nanohelices aligned parallel (top) or orthogonal (bottom) to a light beam. (b) Theoretical calculations. Top: only transverse plasmons are excited if the nanohelices are aligned parallel to the light beam. Bottom: longitudinal (blue) and transverse (red) plasmons are excited if the nanohelices are aligned orthogonal to the light beam. The expected shift of the plasmon resonance is 20.5 nm. (c) Darkfield images of aligned nanohelices in the same area are shown in colour. An ozone-free Xe lamp is used as a light source. (d) The interpolated scattering spectra of a typical nanohelix as highlighted by the white circles inc. Top: the scattering spectrum of a surface-bound nanohelix in solution shows no clear polarization dependency. Only transverse plasmon excitation is obtained (peak indicated by the grey vertical line). Bottom: a dried nanohelix exhibits polarization dependent scattering spectra consistent withxyorientation of the nanohelix. Longitudinal (blue) and transverse (red) plasmon excitation is obtained. The observed shift of the plasmon resonance is 22±4 nm (peaks are indicated by the blue and red vertical lines, respectively). Figure 4c,d shows the darkfield images and scattering spectra of surface-attached L-NHs in solution and dry on a BSA–biotin–neutravidin-functionalized glass slide. For polarization-dependent spectral measurements, the scattered light passes through a linear polarizer before it is fed to a spectrometer. The spectral measurements before and after drying are performed in the same areas and spectra of identical helices are compared. As shown in Fig. 4c , the darkfield image of L-NHs in solution (top) correlates well with that of the same L-NHs after drying (bottom), except for a few unspecifically bound nanohelices that were removed by vigorous rinsing before the nanohelices were dried. For dried L-NHs on glass, the scattering spectra changes with respect to the polarization orientation, as the peak scattering wavelength of the L-NHs depends on the excitable plasmon modes. Here, the peaks for two orthogonal polarizer orientations are separated by 22±4 nm, as shown in Fig. 4d (bottom), consistent with the behaviour of longitudinal and transverse plasmon modes. In contrast, the scattering spectra of L-NHs in solution do not show a clear polarization dependency (top). These experimental results convincingly show agreement with the theoretical predictions (additional darkfield scattering data is shown in Supplementary Figs S10–S14 ). Figure 4: Darkfield scattering spectroscopy of surface-bound nanohelices . Aligned nanohelices orthogonal to a surface in solution (top row) and aligned nanohelices parallel to a surface dry on glass (bottom row) were studied. ( a ) Schemes of nanohelices aligned parallel (top) or orthogonal (bottom) to a light beam. ( b ) Theoretical calculations. Top: only transverse plasmons are excited if the nanohelices are aligned parallel to the light beam. Bottom: longitudinal (blue) and transverse (red) plasmons are excited if the nanohelices are aligned orthogonal to the light beam. The expected shift of the plasmon resonance is 20.5 nm. ( c ) Darkfield images of aligned nanohelices in the same area are shown in colour. An ozone-free Xe lamp is used as a light source. ( d ) The interpolated scattering spectra of a typical nanohelix as highlighted by the white circles in c . Top: the scattering spectrum of a surface-bound nanohelix in solution shows no clear polarization dependency. Only transverse plasmon excitation is obtained (peak indicated by the grey vertical line). Bottom: a dried nanohelix exhibits polarization dependent scattering spectra consistent with xy orientation of the nanohelix. Longitudinal (blue) and transverse (red) plasmon excitation is obtained. The observed shift of the plasmon resonance is 22±4 nm (peaks are indicated by the blue and red vertical lines, respectively). Full size image To summarize, we created a dynamic plasmonic material operating in the visible range by switching of plasmonic chiral nanostructures, which show inverted CD spectra after each switching step. The alignment process leads to a multi-fold increased CD signal over signals resulting from randomly oriented samples at equal concentrations. Switchable chiral nanostructures may be applied as sensors for the detection of molecules, their chirality and their orientation, as systems for data storage and as materials with switchable refractive index. Quartz glass surface preparation A 1 cm by 1 cm quartz slide (CrysTec, Germany) was cut into smaller pieces of ~0.5 cm by 0.5 cm that fit into a cuvette. The pieces were cleaned with Ethanol and placed in a vial (Safe-Lock Tube 2 ml, Eppendorf, Germany) for further treatment. In 1 ml PBS buffer (pH 7.4), 0.8 mg of BSA and 0.2 mg BSA–biotin (both Sigma-Aldrich, Germany) were dissolved. A quartz slide was covered with the BSA-BSA–biotin–PBS solution and incubated overnight at 4 °C (the vial with quartz slides was sealed to prevent drying of the surface). After incubation, the quartz slide was flushed four times with PBS buffer (pH 7.4) in order to remove free BSA–biotin (the surface should not get dry to avoid denaturing of the proteins). In the next step, the quartz slide was covered with the Neutravidin (Thermo Scientific) solution (0.2 mg of Neutravidin per 1 ml PBS buffer (pH 7.4)) for 30 min at 4 °C (Neutravidin binds to the biotin-modified BSA on the surface). Finally, the quartz surface was flushed four times with PBS buffer (pH 7.4) to remove free Neutravidin (the surface should not dry out during this step). Attachment of the nanohelices to the surface Assembly of gold particle nanohelices is described in detail in ref. 2 . Atomic force microscopy imaging of dried L-NH on a quartz surface confirmed the successful assembly ( Supplementary Fig. S15 ). For surface attachment, 50 μl of 4 nM of biotin-modified L-NH in 0.5 × TBE buffer with 11 mM MgCl 2 were added to 600 μl of PBS buffer (pH 7.4). The Neutravidin-coated quartz slide was covered with the nanohelix solution for 2 h at 4 °C. Next, the surface was flushed with 0.5 × TBE+11 mM MgCl 2 buffer in order to remove unbound nanohelices. Metal enhancement of the nanohelices on the quartz surface Equal amounts of the reaction solutions A (initiator), B (moderator) and C (activator) of the HQ Silver Enhancement Kit (nanoprobes.com) were mixed together. One hundred and twenty microlitre of the enhancement kit mix were diluted with 600 μl of 0.5 × TBE+11 mM MgCl 2 buffer. This step should be performed as fast as possible because the enhancement kit becomes active upon mixing of the reaction solutions. The quartz surface with the attached nanohelices was covered with the diluted enhancement solution mix for 4 min. Next the surface was flushed with PBS buffer to stop the enhancement reaction. Efficiency of enhancement depends on the surface density of the nanohelices. Switching the orientation of the nanohelices The switching was performed by direct nitrogen gas flow drying followed by resuspending the gold enhanced nanohelices on the quartz slide in PBS buffer. Gold nanoparticle conjugation to 24HB attached to surface Gold nanoparticles were directly hybridized to the DNA origami structures on the surface. For this, 24HB origami structures with attachment sites for gold nanoparticles were attached to a Neutravidin coated quartz slide. The 24HB coated quartz surface was washed with 0.5 × TBE+11 mM MgCl 2 . Six hundred microlitre of DNA functionalized 10 nm gold nanoparticles (20 nM) in 0.5 × TBE+11 mM MgCl 2 were added to the quartz surface and incubated for 4 h at 20 °C to allow efficient hybridization of gold nanoparticles to the DNA origami structures. Next, the surface was flushed with 0.5 × TBE+11 mM MgCl 2 . After that, the deposition of silver on the gold nanoparticles was performed. Darkfield scattering spectra measurements Optical characterization of the nanohelices was performed to investigate the scattering spectra as a function of nanohelices’ orientation. The glass slide was functionalized with Neutravidin using the protocol described before. The nanohelices were deposited inside the silicone gasket previously applied to the glass surface. A coverslip was immediately placed on top of the gasket and the edges were sealed. The slide was placed on an inverted microscope (Nikon, TiU) upside down (schematic drawing of the setup in Supplementary Fig. S16 ). A xenon lamp (Shutter Instrument model LB-LS/30) illuminates the slide through a high-resolution condenser (Cytoviva). The condenser had a numerical aperture range from 1.2 to 1.4. A × 100 magnification objective (Nikon, Plan Fluor 100 × /0.5–1/3 oil iris) was used to collect the scattering spectra with a 600 lines per mm grating and a CCD camera (Princeton Instruments, ProEM 512). A 480 nm longpass filter (Edmund Optics) was inserted after the lamp to reduce the scattering background generated by the sample substrate. The polarization-dependent scattering spectra were collected for individual nanohelices using a custom-made motorized polarizer, which was inserted into the optical path after the glass slide. The spectrometer’s slit width was set to 30 μm and the camera’s region of interest was set such that only the light emission from the selected nanohelices was collected during the scan from 480 to 760 nm. The exposure time for the CCD camera ranged from 1 to 3 min. To remove background signal that may be present in the scattering spectra, spectra from an adjacent ‘dark’ area containing no sample were subtracted from the scattering spectra. The resulting spectrum was then divided by the spectrum of the xenon lamp. A detailed description of spectral measurements can be found in ref. 43 . After the spectra for nanohelices in buffer solution were characterized, the gasket seal was removed. The glass slide was repeatedly rinsed with buffer solution and passively dried at room temperature. It was then rinsed with milli-Q water to remove salt on the glass surface. The glass slide was loaded back to the microscope. By aligning to the reference marker previously placed on the slide, the same area of the slide where the spectra were taken was located. The reference marker was clearly viewable in the bright field mode on the microscope. How to cite this article: Schreiber, R. et al . Chiral plasmonic DNA nanostructures with switchable circular dichroism. Nat. Commun. 4:2948 doi: 10.1038/ncomms3948 (2013).